Correlated optical and isotopic nanoscopy The isotopic composition of different materials can be imaged by secondary ion mass spectrometry. In biology, this method is mainly used to study cellular metabolism and turnover, by pulsing the cells with marker molecules such as amino acids labelled with stable isotopes ( 15 N, 13 C). The incorporation of the markers is then imaged with a lateral resolution that can surpass 100 nm. However, secondary ion mass spectrometry cannot identify specific subcellular structures like organelles, and needs to be correlated with a second technique, such as fluorescence imaging. Here, we present a method based on stimulated emission depletion microscopy that provides correlated optical and isotopic nanoscopy (COIN) images. We use this approach to study the protein turnover in different organelles from cultured hippocampal neurons. Correlated optical and isotopic nanoscopy can be applied to a variety of biological samples, and should therefore enable the investigation of the isotopic composition of many organelles and subcellular structures. The turnover of subcellular organelles is one of the least understood aspects of modern cell biology, despite its widely recognized importance. In an ideal experiment, the cells are pulsed with specific marker molecules, which are then measured in situ , within various organelles. This type of experiment has not been easy to attempt. For example, radioactivity-based imaging of marker molecules [1] , [2] can only be performed at low-spatial resolution, which precludes the identification of specific organelles. Alternatively, the turnover of single proteins has been investigated by imaging their green-fluorescent-protein-coupled chimeras [3] , [4] , which, however, does not reveal the overall metabolism of the organelles containing the proteins of interest. A different perspective has been introduced by recent improvements in the field of secondary ion mass spectrometry (SIMS) [5] , such as multi-isotope imaging mass spectrometry [6] . In SIMS, the samples are imaged using a primary ion beam, such as Cs + , as a probe. This beam is scanned on the surface of the sample, causing the sputter of secondary particles, atoms or atomic clusters [6] . A proportion of the secondary particles is ionized and can then be identified by mass spectrometry [7] . SIMS has been applied to many types of materials, in different fields of the natural sciences, from geology to soil science and biology. To apply this technology to the study of cellular turnover, the cells are fed with marker molecules that contain stable isotopes such as 15 N and 13 C, which are metabolically incorporated over time. These markers are then imaged with a lateral resolution that depends mainly on the size of the primary ion beam, as the secondary ions are released only from the area exposed to the beam. The resolution has been demonstrated to reach almost 30 nm with modern SIMS instruments such as the Cameca NanoSIMS 50L [6] , [8] , [9] , although the high resolution has generally not always been explicitly indicated in previous publications [10] , [11] , [12] . The z -axis (depth) resolution of SIMS imaging is even higher (as explained below, in the Results). SIMS/multi-isotope imaging mass spectrometry can be used to investigate different cellular structures, as already demonstrated by its application to a number of biological systems, from cell cultures to organisms such as Drosophila and mice [6] , [10] , [11] , [12] , [13] , [14] . Nevertheless, the technique is limited by the fact that specific organelles are not identified with precision. Some structures, such as nuclei, may be identified by their morphology, but this is not the case for most small organelles. To evade this limitation, one would need to combine SIMS with a method that identifies specific organelles. This has not been performed successfully so far. We have addressed this problem here by combining SIMS with fluorescence imaging. We provide a simple protocol that allows samples to be investigated in both SIMS and confocal imaging. Moreover, we have also solved the disparity between the spatial resolution of SIMS and that of conventional microscopy (~200 nm lateral resolution and ~500–600 nm axial resolution) by using super-resolution microscopy (nanoscopy) [15] . The resulting approach, termed correlated optical and isotopic nanoscopy (COIN), allowed us to analyse the turnover for a variety of organelles, and should be easily applied to different biological systems. SIMS and STED provide images with comparable resolution The main difficulty we initially encountered in correlating the SIMS and the microscopy data was to obtain a sufficiently accurate spatial identification of cellular structures. Using conventional microscopy, whose resolution is poorer than that of SIMS, implied that accurately measured isotope positions could not always be placed within their appropriate organelle background. This problem is almost negligible for organelles larger than the diffraction limit, for which we were able to use confocal microscopy. However, small organelles and protein groups can be difficult to discriminate, thus requiring super-resolution microscopy, a group of techniques that provide fluorescence images within or beyond the resolution range of SIMS [16] , [17] ( Supplementary Fig. 1a,b ). To test the feasibility of correlating SIMS with super-resolution microscopy, we turned to stimulated emission depletion (STED). In STED microscopy, the excitation beam is overlaid with a second, toroid-shaped beam that quenches the fluorophores by stimulated emission [18] , [19] . Fluorescence is allowed only at the centre of the excitation beam, resulting in a substantially smaller effective focal spot ( Supplementary Fig. 1c ). The resolution of the technique is no longer limited by diffraction [15] , [18] , and reaches down to at least 50–90 nm ( Supplementary Fig. 1d ) with commercial STED devices [20] and substantially lower values with experimental setups [21] . Protocol for obtaining samples for both SIMS and STED To correlate STED and SIMS images, the biological specimen should be prepared in a form that can be imaged in both setups. The specimen must be stable enough not to suffer any changes between the acquisition of the two images, and it must not be damaged by either of the techniques. As the high-vacuum conditions required for SIMS prohibit the use of live cellular specimens, we decided to fix and embed them in a resin medium that is suitable for multiple microscopy applications. Although SIMS experiments have previously relied on Epon, a resin originally developed for electron microscopy [6] , it cannot be used in correlative imaging due to its high autofluorescence. We therefore replaced Epon with LR White, a polyhydroxy-aromatic acrylic resin with low autofluorescence. For 15 N incorporation, we treated cultured hippocampal neurons [19] with 15 N-labelled leucine for three days. The leucine was incorporated into all the newly produced neuronal proteins, and thus served as a marker for the turnover of neuronal structures. On the fourth day, we fixed the cells and immunostained them for several organelle markers, including the endoplasmic reticulum (ER), the Golgi apparatus, mitochondria and synaptic vesicles. The cells were then embedded in LR White resin according to a protocol we optimized for the best fluorescence and morphology preservation (presented in detail in the Methods). Sections of 200 nm were cut using an ultramicrotome and were deposited on silicon wafers [10] , using procedures that have been standardized for electron microscopy [22] . The use of ultrathin sections, as opposed to whole cells grown on the wafers, has the advantage of increasing the resolution of fluorescence imaging along the vertical axis (otherwise the z -axis resolution of the typical STED microscope is comparable to that of confocal instruments, about 500–600 nm). For correlated imaging, we first investigated the samples using STED microscopy. As the silicon wafers do not allow the transmission of light, we placed the wafers upside-down on the objective stage, with the sections facing the lens, bathed in immersion oil ( Supplementary Fig. 1c ). This procedure did not harm the samples and allowed efficient excitation (using a 635 nm pulsed laser, Leica Microsystems) and fluorescence depletion (using a Mai Tai laser tuned to 750 nm; Supplementary Fig. 1c ). As the exact location of the area imaged by STED needs to be known when the sample is transferred to the SIMS instrument, one needs to create several location markers on the specimen. We achieved this by scanning the regions surrounding the imaged area with the multiphoton beam of the Mai Tai laser at maximum energy. This induced rapid (30–60 s) deformation of the LR White resin, selectively in the regions scanned (see Supplementary Fig. 2 ). Markings of different shapes and sizes can be created around the different areas imaged with STED, allowing easy recognition in the SIMS instrument. The samples were then mounted into a SIMS instrument (NanoSIMS 50L, Cameca). A Cs + beam raster was scanned over the sample surface, applying a sufficient dose of primary ions to reach the steady-state of secondary ion formation. These ions were then mass separated and detected by using a double focalization mass spectrometer (see the Methods for details). Before dealing with biological investigations, we verified the maximum resolution achievable with the SIMS instrument, under our imaging conditions. We imaged gold particles placed in a thin layer of gelatin, as they provide an excellent signal-to-noise [23] . This approach allowed us to verify that a full-width-at-half-maximum of ~50 nm can be regularly achieved for these particles ( Fig. 1a,b ; see also Lechene et al . [6] ). A different definition for the image resolution has often been used in SIMS: the distance across which the signal drops from 84 to 16% of the maximum [6] , [24] . This indicates an even higher resolution for our gold particle images, ~33 nm, or close to the maximum reported with the type of instrument we used [6] , [10] , [11] , [12] . 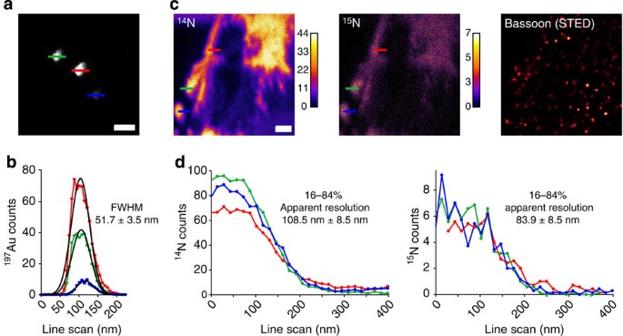Figure 1: The lateral resolution of SIMS imaging in neuronal samples. (a) As a proof-of-principle experiment, upper surfaces of 100 nm gold particles embedded in gelatin were scanned by SIMS. Three particles are indicated. Scale bar, 200 nm. (b) The line scans from panelaare plotted. Gaussian fits to the line scans provide a full-width-at-half-maximum of ~50 nm. The use of a different definition for the image resolution, the signal drop from 84 to 16% of the maximum (which has been frequently used for SIMS6,24) indicates an even higher resolution, of ~33 nm. (c) SIMS analysis:14N and15N images from an axonal area. A STED image of this area shows the immunolabelling for the active zone marker protein bassoon. The STED image was processed with deconvolution. Scale bar, 500 nm. (d) Line scans were performed on the SIMS images from panelc, in the areas indicated by the coloured bars. The resolution, calculated using the 16–84% criterion, is shown as an average of the three line scans±s.d. Figure 1: The lateral resolution of SIMS imaging in neuronal samples. ( a ) As a proof-of-principle experiment, upper surfaces of 100 nm gold particles embedded in gelatin were scanned by SIMS. Three particles are indicated. Scale bar, 200 nm. ( b ) The line scans from panel a are plotted. Gaussian fits to the line scans provide a full-width-at-half-maximum of ~50 nm. The use of a different definition for the image resolution, the signal drop from 84 to 16% of the maximum (which has been frequently used for SIMS [6] , [24] ) indicates an even higher resolution, of ~33 nm. ( c ) SIMS analysis: 14 N and 15 N images from an axonal area. A STED image of this area shows the immunolabelling for the active zone marker protein bassoon. The STED image was processed with deconvolution. Scale bar, 500 nm. ( d ) Line scans were performed on the SIMS images from panel c , in the areas indicated by the coloured bars. The resolution, calculated using the 16–84% criterion, is shown as an average of the three line scans±s.d. Full size image Measurements of SIMS resolution in COIN samples Gold particles have been employed in the study of cellular endocytosis (see for example, Wedlock et al . [23] , but are not typical biological markers. We therefore proceeded to check the SIMS resolution in neuronal sections ( Fig. 1c,d ), prepared as indicated above. Nitrogen was detected in the form of CN − ions (we detected 12 C 14 N − and 12 C 15 N − separately). Figure 1c and Supplementary Fig. 1a show example images for 12 C 14 N − and 12 C 15 N − (labelled, for simplicity, as 14 N and 15 N throughout the text and figures). The lower signal-to-noise ratios inherent to biological samples reduced the performance of the SIMS imaging, but nevertheless resulted in a resolution of ~100 nm or less for both the 14 N and 15 N images ( Fig. 1c,d ). Having established that the lateral resolution of our SIMS images can reach below the resolution of confocal microscopy, we next investigated the z -axis (depth) resolution of the measurements. It has been claimed in the past that the mean penetration depth of the primary ions should be the standard for the axial resolution [25] . However, secondary ions have been shown to be released from shallower depths than the penetration depth of the primary ions [26] . This led to the following definition of the depth resolution of SIMS: ‘the minimum amount of material that needs to be sputtered to obtain an atomic mass image’, which can be as small as ~1 nm [6] . In practice, the amount of sputtered material depends on the sample and on the imaging conditions. To study this in our samples, we collected SIMS images repeatedly in a small area of a neuronal cell body, until the secondary particle generation consumed the sample ( Fig. 2a ). The 200 nm-thick sample was eroded within ~35 SIMS images, indicating that, on average, 5.7-nm-thick sections of the sample were eroded for each image. According to the definition indicated above, the depth resolution of our images would be approximately 5.7 nm. 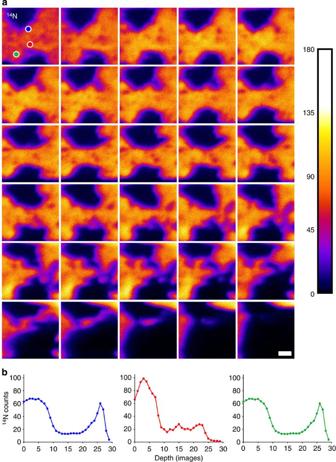Figure 2: The depth resolution of SIMS imaging in neuronal samples. (a) SIMS images were collected repeatedly in one neuronal area. The sample is slowly eroded, which allows the production of images from progressively deeper layers. AZ-stack of the sample is obtained. For simplicity, only the14N images are shown. The 200-nm-thick sample was eroded over 35 images, which indicates that, on average, a sample layer of 5.7 nm is eroded for each image. Scale bar, 500 nm. (b) We analysed the signal changes in three areas, indicated by the coloured circles in the first image in panela(for clarity, the circles are omitted in the following images). Circular regions of interest were used, with a diameter of 152 nm (20 pixels). The signal intensity for each of the three regions of interest (ROI) is shown (averaged for all pixels in each circular regions of interest). Signal changes occur over 2–4 SIMS images. Therefore, according to the 16–84% criterion, the depth resolution is (at most) 11.4–23 nm (as individual images correspond to a depth of 5.7 nm, as indicated above). Figure 2: The depth resolution of SIMS imaging in neuronal samples. ( a ) SIMS images were collected repeatedly in one neuronal area. The sample is slowly eroded, which allows the production of images from progressively deeper layers. A Z -stack of the sample is obtained. For simplicity, only the 14 N images are shown. The 200-nm-thick sample was eroded over 35 images, which indicates that, on average, a sample layer of 5.7 nm is eroded for each image. Scale bar, 500 nm. ( b ) We analysed the signal changes in three areas, indicated by the coloured circles in the first image in panel a (for clarity, the circles are omitted in the following images). Circular regions of interest were used, with a diameter of 152 nm (20 pixels). The signal intensity for each of the three regions of interest (ROI) is shown (averaged for all pixels in each circular regions of interest). Signal changes occur over 2–4 SIMS images. Therefore, according to the 16–84% criterion, the depth resolution is (at most) 11.4–23 nm (as individual images correspond to a depth of 5.7 nm, as indicated above). Full size image An alternative definition of z -axis (depth) resolution has also been made in the past: ‘the depth interval over which the secondary ion intensity drops from 84 to 16% of the maximum [24] ’. According to this definition, a depth resolution of ~14.3 nm was calculated in the past for the NanoSIMS 50 instrument [24] (the same type that we used here). In our samples, the drop in secondary ion ( 14 N) intensity takes place typically over 2–4 SIMS images ( Fig. 2b ), indicating a depth resolution of ~11.4–23 nm, far higher than the axial resolution of fluorescence imaging. COIN imaging of neuronal axons To test the usefulness of combining SIMS with fluorescence imaging, we produced several COIN images. We analysed the enrichment of 15 N at different locations in the neurons, such as axonal areas ( Fig. 3 ) or the cell body ( Fig. 4 ) by calculating the ratio between 15 N and 14 N at different regions of the cell. As in images obtained in the past in comparable experiments [10] , [11] , [12] the ratio, and therefore the relative incorporation of 15 N, is variable in different regions of the cell (close to ~3–8% of all nitrogen atoms, on average, which suggests a high enrichment in comparison to the terrestrial ratio of 0.367% [6] ). 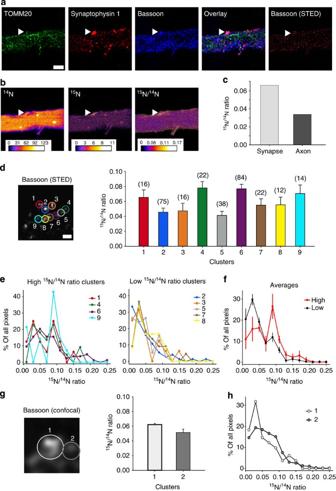Figure 3: Correlated STED and SIMS imaging in neuronal axons. (a) Light microscopy images of a neuronal axon section. The neuron was immunostained for the mitochondrial marker TOMM20 (green, confocal), for the synaptic vesicle marker synaptophysin 1 (red, confocal), and for the active zone marker bassoon (blue, confocal). The overlay of three confocal images is shown. Bassoon staining was also imaged using STED microscopy. All images were processed by deconvolution. Arrowheads indicate a synapse, where all three labels colocalize. Scale bar, 2 μm. (b) SIMS images of the same axon for14N,15N and15N14N ratio, respectively. Note the high15N/14N ratio in the synapse region identified by immunostainings (arrowhead). The natural terrestrial ratio is 0.00367 (ref.6). (c) The bars indicate the15N/14N ratios in the synapse region indicated above and in the rest of the axon, respectively. (d) A high-zoom view of the synapse region in the STED channel. Different clusters of bassoon molecules identified within the synapse are numbered 1 to 9. Their respective15N/14N average ratio values (+s.e.m.) are plotted in the graph. Numbers in parentheses indicate the number of pixels in each cluster. Note that four of the nine clusters have higher ratios (>0.065), while the other ones have lower ratios (~0.055). (e,f) The panel shows the histograms of the clusters in paneld. A K-means clustering approach (performed in Matlab) confirmed that the low- and high-ratio clusters build two different groups. This can also be conformed by inspecting the average histograms for the two groups of clusters (f). The difference between the means of the two groups is statistically significant (t-test,P=0.00078). Scale bar, 250 nm. (g) The clusters indvisualized in confocal mode. Only two clusters can be identified, with relatively similar15N/14N ratios. (h) The histograms for the two confocal clusters ing. Figure 3: Correlated STED and SIMS imaging in neuronal axons. ( a ) Light microscopy images of a neuronal axon section. The neuron was immunostained for the mitochondrial marker TOMM20 (green, confocal), for the synaptic vesicle marker synaptophysin 1 (red, confocal), and for the active zone marker bassoon (blue, confocal). The overlay of three confocal images is shown. Bassoon staining was also imaged using STED microscopy. All images were processed by deconvolution. Arrowheads indicate a synapse, where all three labels colocalize. Scale bar, 2 μm. ( b ) SIMS images of the same axon for 14 N, 15 N and 15 N 14 N ratio, respectively. Note the high 15 N/ 14 N ratio in the synapse region identified by immunostainings (arrowhead). The natural terrestrial ratio is 0.00367 (ref. 6 ). ( c ) The bars indicate the 15 N/ 14 N ratios in the synapse region indicated above and in the rest of the axon, respectively. ( d ) A high-zoom view of the synapse region in the STED channel. Different clusters of bassoon molecules identified within the synapse are numbered 1 to 9. Their respective 15 N/ 14 N average ratio values (+s.e.m.) are plotted in the graph. Numbers in parentheses indicate the number of pixels in each cluster. Note that four of the nine clusters have higher ratios (>0.065), while the other ones have lower ratios (~0.055). ( e , f ) The panel shows the histograms of the clusters in panel d . A K-means clustering approach (performed in Matlab) confirmed that the low- and high-ratio clusters build two different groups. This can also be conformed by inspecting the average histograms for the two groups of clusters ( f ). The difference between the means of the two groups is statistically significant ( t -test, P =0.00078). Scale bar, 250 nm. ( g ) The clusters in d visualized in confocal mode. Only two clusters can be identified, with relatively similar 15 N/ 14 N ratios. ( h ) The histograms for the two confocal clusters in g . 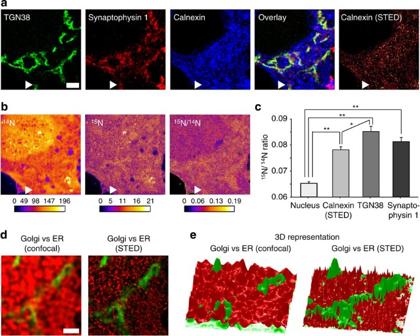Figure 4: Correlated STED and SIMS imaging in neuronal cell bodies. (a) Light microscopy images of a neuronal cell body section. The neuron was immunostained for the Golgi marker TGN38 (green, confocal), for the synaptic vesicle marker synaptophysin 1 (red, confocal; synaptophysin 1 identifies vesicle precursors in the cell body), and for the ER marker calnexin (blue, confocal). The overlay of three confocal images is shown. Calnexin staining was also imaged using STED microscopy. All images were processed by deconvolution. Scale bar, 2 μm. (b) SIMS images for14N,15N and15N/14N ratio, respectively. Note the low15N/14N ratio in the nucleus (which is identified by its characteristic morphology, upper left corner of the image) and the presence of several cytosolic regions with higher ratios. (c) The graph shows the15N/14N ratio for the different organelles. The values for the nucleus are significantly lower than those for all the other organelles (**,P<0.01,t-test). In addition, the ratio is significantly higher in the Golgi apparatus (TGN38) than in the ER (calnexin; *,P<0.05,t-test). The graphs represent mean+s.e.m., from 26, 57, 9, and 41 regions for the four bars, respectively. For each set of data we performedt-tests of the null hypothesis that data analysed were random samples from a normal distribution. The tests did not disprove the hypothesis (P=1). Sample variance was low: 1.16 × 10−5, 7.55 × 10−5, 3.57 × 10−5, 10.49 × 10−5for the four bars, respectively. (d,e) Comparison between the ability of confocal and STED microscopy to determine accurate organelle outlines. The panels show an overlay of the Golgi apparatus (green) with the ER (red) in confocal imaging or in STED imaging, as double-coloured images (d) and as 3D views (e). Scale bar, 1 μm. The confocal image of the ER overlaps more extensively with that of the Golgi in comparison to the STED image. Therefore, correlation with STED enables much more accurate identification of the ER-free Golgi areas and allows measurement of the associated15N signal. This suggests that SIMS measurements based on the STED image are more precise than those based on the confocal images. See alsoSupplementary Fig. 7for a modelling study confirming this aspect. Full size image Figure 4: Correlated STED and SIMS imaging in neuronal cell bodies. ( a ) Light microscopy images of a neuronal cell body section. The neuron was immunostained for the Golgi marker TGN38 (green, confocal), for the synaptic vesicle marker synaptophysin 1 (red, confocal; synaptophysin 1 identifies vesicle precursors in the cell body), and for the ER marker calnexin (blue, confocal). The overlay of three confocal images is shown. Calnexin staining was also imaged using STED microscopy. All images were processed by deconvolution. Scale bar, 2 μm. ( b ) SIMS images for 14 N, 15 N and 15 N/ 14 N ratio, respectively. Note the low 15 N/ 14 N ratio in the nucleus (which is identified by its characteristic morphology, upper left corner of the image) and the presence of several cytosolic regions with higher ratios. ( c ) The graph shows the 15 N/ 14 N ratio for the different organelles. The values for the nucleus are significantly lower than those for all the other organelles (**, P <0.01, t -test). In addition, the ratio is significantly higher in the Golgi apparatus (TGN38) than in the ER (calnexin; *, P <0.05, t -test). The graphs represent mean+s.e.m., from 26, 57, 9, and 41 regions for the four bars, respectively. For each set of data we performed t -tests of the null hypothesis that data analysed were random samples from a normal distribution. The tests did not disprove the hypothesis ( P =1). Sample variance was low: 1.16 × 10 −5 , 7.55 × 10 −5 , 3.57 × 10 −5 , 10.49 × 10 −5 for the four bars, respectively. ( d , e ) Comparison between the ability of confocal and STED microscopy to determine accurate organelle outlines. The panels show an overlay of the Golgi apparatus (green) with the ER (red) in confocal imaging or in STED imaging, as double-coloured images ( d ) and as 3D views ( e ). Scale bar, 1 μm. The confocal image of the ER overlaps more extensively with that of the Golgi in comparison to the STED image. Therefore, correlation with STED enables much more accurate identification of the ER-free Golgi areas and allows measurement of the associated 15 N signal. This suggests that SIMS measurements based on the STED image are more precise than those based on the confocal images. See also Supplementary Fig. 7 for a modelling study confirming this aspect. Full size image First, we targeted several organelles of the synapse ( Fig. 3a ). The synapse contains neurotransmitter-filled synaptic vesicles, which release their contents by fusing to the plasma membrane at specific sites termed active zones. We identified synaptic vesicles by immunostaining for synaptophysin 1, one of their most important components; similarly, active zones were detected by staining for one of their major proteins, bassoon [27] . We also identified mitochondria, which deliver the energy necessary for synaptic transmission, by staining for the mitochondrial transport protein TOMM20. Figure 3a shows a section through a neuronal branch (axon) in which a synapse, characterized by the colocalization of all three types of organelles (vesicles, active zone, mitochondria), is indicated by the white arrowheads. The rest of the cytosol was populated by numerous transport vesicles containing synaptophysin 1 or bassoon, and by several other mitochondria. The turnover of this synapse appears to have been stronger than that of the neighbouring axon, as the synapse contained higher levels of 15 N-leucine ( Fig. 3b,c ). The resolution of the SIMS images is indicated by line scans shown in Supplementary Fig. 3a . Supplementary Fig. 3b,c also presents the line scans performed in the correlated fluorescence and SIMS images, showing the overlap of different organelles (identified by fluorescence microscopy) with the metabolic labels ( 14 N, 15 N). Interestingly, the edges of the axon appear somewhat blurry in the SIMS image. An electron microscopy investigation ( Supplementary Fig. 4 ) suggests that this is likely due to the presence of protein-rich material on the outside of the cell, probably in the form of extracellular matrix components. We used confocal imaging for both TOMM20 and synaptophysin 1, and STED imaging for bassoon. Confocal imaging allowed the identification of organelles in the general synaptic area, and even allowed separating the mitochondria from the synaptic vesicle cluster [27] . This is possible as both mitochondria and the vesicle cluster are larger than the diffraction limit. However, the advantage of STED imaging is evident when groups of bassoon molecules, which are much smaller than the diffraction limit, are investigated ( Fig. 3d–f ). The synaptic area contained several groups of bassoon molecules, four of which presented much higher incorporation of 15 N-leucine than the others. This level of detail is invisible with conventional microscopy ( Fig. 3g,h ). The presence of two groups of bassoon clusters, with low and high turnover rates ( Fig. 3e,f ), demonstrates that newly synthesized protein clusters coexist with older structures within single synapses. This confirms that the material in synaptic boutons is replaced gradually over time, as often hypothesized in the past [28] . A thorough future study of the replacement of different synaptic organelles (synaptic vesicles, endosomes, mitochondria, active zone components) will provide substantial new information on the metabolic rates of individual synapses. COIN imaging of turnover in the cell body of neurons We also investigated organelles in the neuronal cell body, a typical example of which is shown in Fig. 4a,b . We immunostained for the trans-Golgi marker TGN38 and for synaptophysin 1, a marker of synaptic vesicle precursors, as well as for the ER marker calnexin. Confocal imaging was applied for TGN38 and synaptophysin 1, while the denser calnexin labelling was imaged by STED. The nucleus, easily identified by its morphology, had the lowest incorporation of 15 N-leucine of all identifiable organelles ( Fig. 4c ). In contrast, the trans-Golgi network (TGN38 bar) contained high levels of newly produced proteins, as did the synaptic vesicle precursors (synaptophysin 1 bar); note that synaptic vesicle precursors overlapped partially with both the Golgi and the ER. Interestingly, the ER (calnexin bar) contained a much lower proportion of new proteins than the trans-Golgi, suggesting that newly produced proteins leave the ER rapidly, but linger substantially longer in the Golgi apparatus (see also Supplementary Fig. 5 , for an analysis of the resolution of the SIMS images, and for a line scan-based evaluation of the image correlation). Although these measurements seem appropriate for large organelles such as the nucleus and the Golgi apparatus, confocal imaging is no longer sufficient for the diffuse, high-density calnexin staining. It is extremely difficult to determine which parts of the Golgi apparatus are free from overlap with the ER staining based on the confocal images ( Fig. 4d,e ). This is easily achieved by STED imaging ( Fig. 4d,e ), suggesting that correlation with super-resolution microscopy is necessary for studying small or densely packed organelles. Overall, these experiments indicate that COIN is a feasible approach. Each of the two combined technologies provides a piece of information that is unavailable for the other: SIMS yields the isotopic composition of the material investigated, and even its turnover (as indicated by the 15 N/ 14 N ratio), while STED microscopy reveals the identities and the spatial distribution of organelles or organelle components. An important note of caution is, however, linked to the sample preparation, as inaccurate fixation, immunostaining and/or embedding might induce misleading results. An overview of the parameters we optimized in order to obtain efficient stainings without compromising structure preservation is presented in Supplementary Discussion . The use of COIN in conjunction with high-pressure freezing and freeze-substitution, which would ensure even higher cellular preservation, is conceivable in the future. One difficulty that may be apparent for fluorescence microscopy specialists is that our SIMS images are far noisier than the fluorescence images. This could be addressed, to some extent, by accumulating a series of SIMS images ( Supplementary Fig. 6 ). However, the noise of SIMS images, as presented here, is due to the inherent noisy nature of metabolic (bulk) 15 N incorporation, and not due to difficulties with SIMS imaging (as demonstrated by modelling SIMS versus fluorescence imaging, Supplementary Fig. 7a–f ). Depending on how labelling is achieved, SIMS can deliver images with much lower levels of noise (see gold particle images in Fig. 1 ). Despite the higher noise associated with metabolic labelling, averaging the SIMS signal over different areas does provide reliable results ( Supplementary Fig. 7g ). In the past, the investigators defined such areas only by following the morphology of the preparation. COIN imaging now enables us to define areas of interest based on the correlated fluorescence images. Our modelling approach demonstrates that defining such an area based on STED imaging provides a far higher precision for the SIMS measurements than the use of confocal imaging ( Supplementary Fig. 7g ). We suggest that COIN has a large field of potential applications, as it enables the investigation of the metabolism and organization of any cellular organelle. This is not restricted to the analysis of nitrogen or carbon isotope ratios. Many other cellular isotopes can be analysed (such as Si, S, As, P), which may be of interest especially in plant or bacterial biology [29] . Finally, a further potential use of this procedure is the generation of triple-correlation images, as the samples prepared for COIN can also be investigated with scanning electron microscopy [30] , thus allowing a combination of super-resolution fluorescence microscopy, electron microscopy and SIMS on the same sample. Sample preparation Primary cultures of hippocampal neurons (prepared from new-born rats, plated onto astrocytic monolayers [19] and used after 10 days in vitro ) were incubated in Neurobasal-A medium (GIBCO) with 2% B27 Supplement (GIBCO), 1% GlutaMAX Supplement (GIBCO) and 60 units ml −1 Penicillin–Streptomycin (Lonza) in the presence of 2.2 mM 15 N-leucine for 3 days. The cells were fixed for with 4% paraformaldehyde in phosphate-buffered saline (PBS) for 15 min on ice followed by 30 min at room temperature, and quenched for 25 min with 100 mM NH 4 Cl. Then permeabilization and blocking was performed with 0.1% Triton-X100 in PBS containing 1.5% bovine serum albumin for 15 min at room temperature. The cells were incubated for 1 h at room temperature with the following primary antibodies: for Figs 1 and 3 , mouse monoclonal anti-TOMM20 (Sigma, WH0009804M1), guinea pig synaptophysin 1 (Synaptic Systems, 101004) and rabbit polyclonal anti-bassoon (Synaptic Systems, 141002); for Fig. 4 , mouse monoclonal anti-TGN38 (BD Biosciences, 610898), guinea pig synaptophysin 1 (Synaptic Systems, 101004) and rabbit polyclonal anti-calnexin (Abcam, 22595). Primary antibodies were detected using goat anti-mouse Cy2 (Dianova, 115-225-146), donkey anti-guinea pig Cy3 (Dianova, 706-165-148) and Atto647N-labelled goat anti-rabbit (Rockland, 611-156-122S). After washing, a post-fixation step was performed with 4% paraformaldehyde and 0.2% glutaraldehyde in PBS for 30 min at room temperature, followed by quenching with 100 mM NH 4 Cl in PBS for 15 min. The optimization of the immunostaining protocol is discussed in detail in Supplementary Discussion . Gold particles used for Fig. 1 and Supplementary Fig. 4 were purchased from Sigma Aldrich. Embedding First partial serial dehydration was performed with ethanol: 30% ethanol for 5 min, three times 50% ethanol for 5 min each, and incubation with 1:1 mixture of 50% ethanol and LR White (London Resin Company Ltd) for 30 min. This was followed by the incubation of coverslips with LR White in ethanol-free conditions for 1 h. The cells were then embedded at 4 °C with LR White and accelerator mixture (London Resin Company Ltd), and incubated for 15 min. Later, they were incubated for 90 min at 60 °C, and cooled down to room temperature. 200-nm-sections were cut from the resulting blocks using an EM UC6 ultramicrotome from Leica Microsystems. Fluorescence imaging Fluorescence images were acquired using a Leica TCS SP5 STED confocal microscope (Leica Microsystems) equipped with a 100 × 1.4N.A. HCX PL APO CS oil objective (Leica) and the Leica Application Suite Advanced Fluorescence software. In STED mode, the excitation of Atto647N was performed using a pulsed diode laser (Leica Microsystems) at 635 nm, and depletion was achieved by means of a Spectra-Physics Mai Tai tunable laser (pulsed at 80 MHz; Titanium Sapphire, Newport Spectra-Physics) at 750 nm, with an output power of 1.6 W. For multichannel confocal images, the following excitation lines were used: an argon laser at a wavelength of 488 nm and Helium-Neon lasers at 594 nm and 633 nm, for the Cy2, Cy3, and Atto647 channels, respectively. Appropriate emission intervals were selected using an AOTF filter (Leica) and line-by-line sequential scanning at 1,000 Hz was applied with 32 times line averaging for confocal and 96 times line averaging for STED. Images of 2,048 × 2,048 pixels were taken at × 3 zoom at a final pixel size of 25.2 nm. Signal detection was performed using photomultiplier tubes in confocal mode and an avalanche photodiode in STED mode. SIMS imaging SIMS imaging was performed by using a Cameca NanoSIMS 50L instrument from Cameca (France). A 133 Cs + primary ion beam at 16 keV energy was used to sputter and partly ionize atoms belonging to the sample. These ions were then mass separated and detected by using a double focalization mass spectrometer equipped with seven miniature electron multipliers (Hamamatsu). The mass resolving power was adjusted to suppress interferences at all masses (allowing the optimal separation of 12 C 15 N − from interfering ions like 13 C 14 N − ). Primary ion beam current was 0.5 to 1 pA, scanning parameters were 512 × 512 pixels for areas of 3.2 to 12.9 μm with a dwell time of 500 μs per pixel. All figures represent data from single plane without accumulation. Image processing For Figs 1 , 3 and 4 , the fluorescence images were rotated and aligned to the SIMS images. A background subtraction was performed for the 15 N/ 14 N ratio images, for display purposes. All line scans and spot size measurements were performed using custom-written routines in MATLAB (The Mathworks Inc). Only horizontal line scans were used; several lines were averaged, to increase the signal-to-noise ratio (three lines for Fig. 1a and Supplementary Fig. 1 ; 5 lines for Supplementary Figs 3b and 5b ; three lines for all other 14 N images, and seven lines for all other 15 N images, unless otherwise noted in the figure legends). Fluorescence images were deconvolved (applying classical maximum likelihood estimation algorithm) with the aid of Huygens Essential software (Scientific Volume Imaging), using the inbuilt routines designed specifically for confocal and STED images. For identifying individual protein clusters in Fig. 3 , we first selected a region of interest centred on the synapse (indicated by an arrowhead in Fig. 3a ). The region was then filtered using a median filter (2 × 2 pixels), to remove noise. The resulting image was then thresholded using an empirically derived threshold, equivalent to the mean intensity of the regions of interest plus two to ten arbitrary units (depending on the image). The thresholding was applied at the pixel level (not at subpixel levels), and resulted in separated regions of interest corresponding to the individual protein clusters. These were subsequently analysed as indicated in the main text and in Fig. 3 . How to cite this article: Saka, S. K. et al. Correlated optical and isotopic nanoscopy. Nat. Commun. 5:3664 doi: 10.1038/ncomms4664 (2014).